Protein interaction network of alternatively spliced isoforms from brain links genetic risk factors for autism Increased risk for autism spectrum disorders (ASD) is attributed to hundreds of genetic loci . The convergence of ASD variants have been investigated using various approaches, including protein interactions extracted from the published literature. However, these datasets are frequently incomplete, carry biases and are limited to interactions of a single splicing isoform, which may not be expressed in the disease-relevant tissue. Here we introduce a new interactome mapping approach by experimentally identifying interactions between brain-expressed alternatively spliced variants of ASD risk factors. The Autism Spliceform Interaction Network reveals that almost half of the detected interactions and about 30% of the newly identified interacting partners represent contribution from splicing variants, emphasizing the importance of isoform networks. Isoform interactions greatly contribute to establishing direct physical connections between proteins from the de novo autism CNVs. Our findings demonstrate the critical role of spliceform networks for translating genetic knowledge into a better understanding of human diseases. Autism spectrum disorder (ASD) is a broad class of neurodevelopmental disorders with a common set of core features including social impairments, communication difficulties and repetitive behaviours. The genetic aetiology of ASDs is also highly heterogeneous and can be attributed to hundreds of genes, of which only a small fraction have sufficient genetic evidence to be considered as causative. Some of the most well-documented autism risk factors include genes associated with rare syndromic forms of ASD ( MECP2, FMR1, PTEN ), synaptic cell adhesion and scaffolding molecules (NLGN3, NLGN4, NRXN1, CNTNAP2, SHANK3) and genes with de novo mutations ( CHD8, SCN2A, DYRK1A among others) recently identified in exome-sequencing studies [1] , [2] , [3] , [4] . Copy number variation (CNV) [5] , [6] , [7] and genome-wide association studies [8] , [9] , [10] have discovered rare and common variants, respectively, that confer varying effects on ASD risk in the general population. The heterogeneity of genes implicated in ASD stimulated intensive testing of the pathway convergence hypotheses [11] . The experimental and computational approaches including gene coexpression [12] , [13] , functional annotations [14] , [15] , mouse model phenotypes [16] and protein–protein interactions (PPIs) [3] , [17] , [18] were used to search for molecular processes and pathways shared by the ASD risk factors. With regard to convergence at the protein interactions level, only one experimental PPI study of 35 syndromic ASD genes is currently available [17] ; all other PPI studies in ASD to date have been based on the interactions extracted from the published literature. However, literature PPI datasets are known to be incomplete and inherently biased [19] . For example, the largest database of autism candidate genes, ‘Simons foundation autism research initiative (SFARI) gene’ ( https://sfari.org/resources/sfari-gene ), contains human binary physical protein interaction annotations for only 24% (131/546, June 2013 release) of its entries. The annotations of interactions between ASD genes, which is even more important for discovering the desired convergence, is scarcer still—only 9% (50/546) of SFARI proteins are annotated as interacting with each other. In addition, literature interactions carry a wide range of other biases: highly studied proteins have a greater number of interactions, computationally predicted, erroneously annotated and non-binary interactions may be included in the analyses [19] , [20] . Most importantly, the interactions of the alternative splice forms of genes have not been systematically incorporated into disease networks, even though most human genes are alternatively spliced [21] , [22] . Historically, only a single so-called ‘reference’ isoform of each gene (or its fragments) has been used in the disease PPI network studies [17] , [23] , [24] , [25] . Here we apply a novel approach to mapping an ASD interactome network by experimentally testing multiple naturally occurring brain-expressed alternatively spliced isoforms of nearly 200 autism candidate genes for interactions. In addition, we also test all cloned splicing isoforms of these genes for interactions against themselves and identify important novel PPIs between variants of the ASD risk factors. We demonstrate that the resulting Autism Spliceform Interaction Network (ASIN) provides greater detail and depth around ASD proteins than the conventional PPI networks. ASIN directly connects genes from a large number of ASD-relevant CNVs into a single connected component. We identify two proteins as important connectors between CNV loci , and implicate new players in ASD. Overall, our isoform-based autism interactome provides the detailed and unprecedented look at the cellular network involving a large number of ASD risk factors. Constructing autism brain-expressed isoform ORF library To obtain a network of physical interactions between proteins implicated in autism, we performed global interactome mapping for 191 autism candidate genes and their cloned brain-expressed splice variants ( Fig. 1a ). The list of selected ASD risk factors (Methods, Supplementary Data 1 ) consisted of genes associated with syndromic forms of ASD (for example, TSC2 and FMR1; a total of 24); genes affected by the de novo CNVs (for example, ARID1B and A2BP1 also known as RBFOX1; a total of 65) or recurrent CNVs (for example, PTCHD1 and CNTN4; a total of 27); genes carrying rare mutations in autism patients (for example, SCN2A and GRIN2A; a total of 25), and genes with suggestive evidence for association with autism (for example, CDH9 and CDH10; a total of 50). Recently, a rapidly growing number of genes have been implicated in ASD with varying degrees of confidence: from very strong for a handful of the syndromic genes to suggestive for hundreds of genes from the CNV and the genetic-association studies. As a result, an attempt to prioritize ASD candidate genes is inevitably subjected to a range of biases. Here, we decided to create a broad list of non-syndromic ASD candidates by including all genes with suggestive evidence that were available in the published literature at the time when this study began (early 2010), in addition to the genes with strong evidence from the syndromic ASD studies. Since our study began before the publication of ASD exome sequencing studies [1] , [2] , [3] , [4] , the new genes with de novo mutations identified in these studies were not included in our candidate gene list. 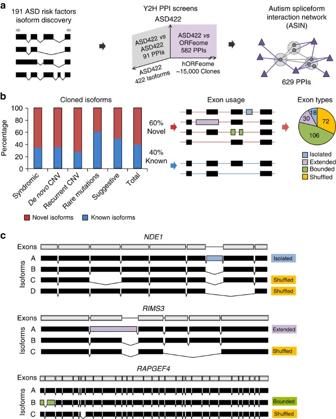Figure 1: Splicing isoform cloning and construction of autism spliceform network. (a) The experimental pipeline used to construct ASIN. High-throughput splice isoform discovery and cloning was performed for 191 ASD risk factors using total RNA purified from the pooled foetal and adult whole brain samples. A total of 422 splicing isoforms of these genes were assayed by Y2H screens for interactions against 15,000 human ORFs (ASD422 versus ORFeome) and against themselves (ASD422 versus ASD422) to construct the ASIN with 629 isoform-level PPIs. (b) Novelty assessment of the discovered splice isoforms. Isoform novelty was evaluated based on the annotations from six public databases. The ratios of known and novel cloned isoforms among different categories of ASD risk factors is uniform, with genes with rare mutations having slightly lower number of cloned novel isoforms. Exons used to generate novel isoforms were assigned in the following order: ‘isolated’, ‘extended’, ‘bounded’ and ‘shuffled’. The majority of novel isoforms were generated using ‘bounded’ exons. (c) The examples of cloned isoforms carrying four types of exons. An intronic region ofNDE1is converted into a coding region (‘isolated’); the exon 2 ofRIMS3is extended with an intronic region (‘extended’); the partial deletion of the first two exons ofRAPGEF4(‘bounded’) and a novel exonic combinations in all three genes (‘shuffled’) are shown. The introns are not to scale. Figure 1: Splicing isoform cloning and construction of autism spliceform network. ( a ) The experimental pipeline used to construct ASIN. High-throughput splice isoform discovery and cloning was performed for 191 ASD risk factors using total RNA purified from the pooled foetal and adult whole brain samples. A total of 422 splicing isoforms of these genes were assayed by Y2H screens for interactions against 15,000 human ORFs (ASD422 versus ORFeome) and against themselves (ASD422 versus ASD422) to construct the ASIN with 629 isoform-level PPIs. ( b ) Novelty assessment of the discovered splice isoforms. Isoform novelty was evaluated based on the annotations from six public databases. The ratios of known and novel cloned isoforms among different categories of ASD risk factors is uniform, with genes with rare mutations having slightly lower number of cloned novel isoforms. Exons used to generate novel isoforms were assigned in the following order: ‘isolated’, ‘extended’, ‘bounded’ and ‘shuffled’. The majority of novel isoforms were generated using ‘bounded’ exons. ( c ) The examples of cloned isoforms carrying four types of exons. An intronic region of NDE1 is converted into a coding region (‘isolated’); the exon 2 of RIMS3 is extended with an intronic region (‘extended’); the partial deletion of the first two exons of RAPGEF4 (‘bounded’) and a novel exonic combinations in all three genes (‘shuffled’) are shown. The introns are not to scale. Full size image Using total RNA (Clontech, Stratagene) purified from the pooled foetal and adult whole brain samples (Methods) and applying a high-throughput isoform discovery pipeline and deep-well next-generation sequencing [26] , we successfully cloned 373 brain-expressed splicing isoforms corresponding to 124 autism candidate genes ( Supplementary Fig. 1 ). To further increase the coverage, the set of cloned isoforms was supplemented with additional open reading frames (ORFs) from the human ORFeome 5.1 (ref. 27 ) resulting in a library of 422 splicing isoforms for 168 genes (ASD422, Fig. 1a , Supplementary Data 2 ). While the isoform space coverage in our study is limited to an average of ~2.5 isoforms per gene, the advantage of our approach lies in the creation of the physical collection of the full-length splicing isoforms that is not available from the RNA-seq studies. By comparing the full-length sequences of the cloned isoforms to the full-length sequences annotated in six public databases (consensus coding sequence (CCDS), RefSeq, GenCode, UCSC, MGS and ORFeome) we observed that over 60% of the cloned isoforms are novel—that is, have not previously been reported in any of these databases ( Fig. 1b ). The distribution of novel and known cloned splicing variants among different subclasses of genes selected for this study was fairly uniform, and only genes with rare mutations had slightly decreased fraction of cloned novel isoforms ( Fig. 1b ). Considering that the brain is among the tissues with the highest frequency of alternative splicing events [22] , the large number of novel isoforms that we cloned was not unexpected. Furthermore, the high fraction of novel brain-expressed isoforms is consistent with a previous study that also identified the highest proportion of novel isoforms in the brain while investigating five different tissue types [26] . We examined the splicing patterns by which novel isoforms were produced. We observed that according to previously introduced classification [21] , most novel isoforms were generated using either ‘bounded’ exons (47%) that contain partial fragments of known exons, or by reshuffling of known exons (32%) ( Fig. 1b ). The remaining isoforms had at least one new exon (8%) that did not overlap with any known exons, or had an ‘extended’ exon (13%) consisting of a known exon extended with the adjacent novel exonic region. The cloned splicing variants of three genes ( NDE1, RIMS3 and RAPGEF4 ) demonstrate that isoforms may carry different types of exons or combinations of exons ( Fig. 1c ). Autism spliceform interaction network To build an autism spliceform interaction network (ASIN), the ASD422 isoform library was tested in two independent high-throughput yeast-two-hybrid (Y2H) screens ( Fig. 1a ). The first screen tested 422 ORFs for interactions against the human ORFeome 5.1 (ref. 27 ) comprising ~15,000 ORFs. The second screen tested interactions among the ASD422 ORFs themselves. Isoform interactions identified in these screens using next-generation sequencing were subsequently confirmed by Sanger sequencing ( Supplementary Fig. 2 , Methods). To increase confidence of detected isoform interactions and to ensure that interaction changes are indeed owing to alternative exon usage by the isoforms, all corresponding protein isoforms for any given gene were Y2H-retested four times in a pair-wise format against the full series of interactors of any protein isoform of that gene found in the primary screens, thereby controlling for potential biases owing to sampling sensitivity (that is, all isoforms against all interaction partners of any isoform of that gene). Only the interactions that scored positive at least three times in the retests were retained, and only those isoforms with at least one interacting partner were used for the subsequent analyses. Finally, the isoforms without any interacting partners were eliminated from the analyses and were not considered as having lost interactions (that is, negatives). We detected 506 positive physical binary PPIs (corresponding to 629 isoform-level PPIs) between 71 baits (autism risk factors) and 291 preys (genes from the human ORFeome collection or from ASD422 isoform library; Supplementary Data 3–5 ). Most (463/506 or 91.5%) of the detected PPIs were novel, based on a comparison with a comprehensive literature-curated interaction dataset (LCI) of over 35,000 high-confident physical binary interactions assembled from seven public databases (MIPS, BIND, DIP, MINT, IntAct, BioGRID and PDB) ( Supplementary Methods ). Validation of ASIN interactions by mammalian PPI trap assay To ensure that we have constructed a high-quality network, 312 interaction pairs corresponding to 62% of gene-level interactions in ASIN were retested in an orthogonal assay, mammalian PPI trap assay (MAPPIT) [28] , and then benchmarked against a positive reference set (PRS) and a random reference set (RRS), consisting of ~500 and ~700 protein pairs, respectively. The ASIN validation set was assembled by following a two-tier procedure (Methods) and consisted of the interacting protein pairs unique at a gene-level but at the same time represented by a diverse set of the isoforms. The validation rate of ASIN interactions was similar to that of PRS ( n ASIN =312 versus n PRS =460, Wilcoxon P =0.85) and was significantly higher than that of RRS ( n ASIN =312 versus n RRS =698, Wilcoxon P =1.78·10 −11 ; Fig. 2a ). The precision of ASIN (89.2%) estimated at the RRS recall rate of 0.01 was comparable to that of two other interactome networks, human (79%) [29] and Arabidopsis (80%) [30] . 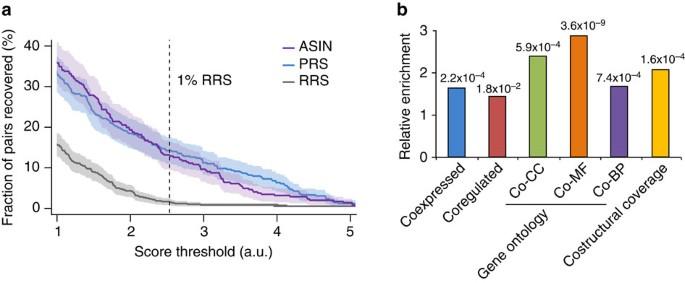Figure 2: Autism spliceform network quality assessment. (a) ASIN validation rate in the orthogonal mammalian system MAPPIT.Y-axis shows the fraction of ASIN, positive reference protein pairs set (PRS) and random reference set (RRS) pairs recovered by MAPPIT at increasing RRS recovery rates; 1% RRS recovery rate is indicated by a vertical dotted line. The shading indicates standard error of the proportion. The validation success rate of ASIN is comparable with the rate of true-positive interactions (nASIN=312 versusnRRS=698P=1.78·10−11;nASIN=312 versusnPRS=460P=0.85;nPRS=460 versusnRRS=698P=8.1·10−12; two-sided Wilcoxon rank sum tests). (b) Interacting ASIN pairs are significantly enriched in coexpressed, coregulated and co-GO-annotated protein pairs, as well as in protein pairs forming binary complexes with experimentally solved or homology-modelled structures. The comparison was performed against the background control dataset that consisted of ~1.2 million non-redundant protein pairs generated by pairing each ASIN protein with each protein from the human ORFeome 5.1.P-values were calculated using one-tailed Fisher’s exact test. Figure 2: Autism spliceform network quality assessment. ( a ) ASIN validation rate in the orthogonal mammalian system MAPPIT. Y -axis shows the fraction of ASIN, positive reference protein pairs set (PRS) and random reference set (RRS) pairs recovered by MAPPIT at increasing RRS recovery rates; 1% RRS recovery rate is indicated by a vertical dotted line. The shading indicates standard error of the proportion. The validation success rate of ASIN is comparable with the rate of true-positive interactions ( n ASIN =312 versus n RRS =698 P =1.78·10 −11 ; n ASIN =312 versus n PRS =460 P =0.85; n PRS =460 versus n RRS =698 P =8.1·10 −12 ; two-sided Wilcoxon rank sum tests). ( b ) Interacting ASIN pairs are significantly enriched in coexpressed, coregulated and co-GO-annotated protein pairs, as well as in protein pairs forming binary complexes with experimentally solved or homology-modelled structures. The comparison was performed against the background control dataset that consisted of ~1.2 million non-redundant protein pairs generated by pairing each ASIN protein with each protein from the human ORFeome 5.1. P -values were calculated using one-tailed Fisher’s exact test. Full size image To confirm the biological relevance of the detected interactions, we also examined coexpression, coregulation and cofunctional annotation of all ASIN protein pairs using Gene Ontology (GO) terms (Methods). Interacting protein pairs from ASIN were significantly enriched in the coexpressed pairs, in the pairs that share transcription factor-binding sites and in the pairs with shared GO terms when compared with random pairs of proteins ( Fig. 2b ). Furthermore, the interacting protein pairs from ASIN formed binary protein complexes with experimentally solved or homology-modelled structures more frequently than random pairs (Methods). High retest rate of ASIN interactions in the mammalian system together with its enrichment in pairs with shared functional annotations and structures suggest that ASIN is a high-quality network of biologically-relevant interactions. Most importantly, ASIN is the first high-resolution disease network built using multiple full-length splicing isoforms of hundreds of genes, all derived from a disease-relevant brain tissue. Splicing isoform interactions expand ASIN Typically, a PPI screen will test only a single ‘reference’ isoform of each gene. We investigated whether additional isoform interactions detected in our study expand this ‘reference’ network and add new isoform-specific PPIs. We constructed the ‘reference’ ASIN network by including only interactions corresponding to a single, ‘reference’ isoform (typically CCDS ORF) of each ASIN gene ( Fig. 3a ). We observed that this ‘reference’ network comprises approximately half of all detected PPIs. The remaining 46% of the isoform-level PPIs, corresponding to 33% of the gene-level PPIs, would not have been identified if we only screened ‘reference’ isoform of each gene for interactions ( Fig. 3b ). Notably, many PPIs that we have identified were derived exclusively from the non-reference isoforms, emphasizing the importance of isoform screening for building more complete PPI networks. 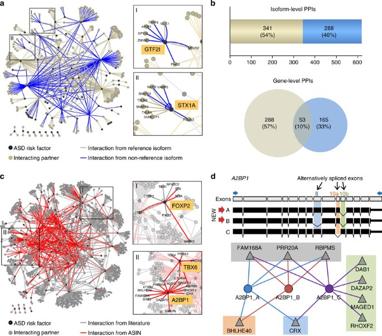Figure 3: Splicing isoform interactions expand ASIN. (a) ASIN represented as two-component network consisting of reference isoforms PPIs (tan edges) and non-reference isoforms PPIs (blue edges). The network represents an isoform-level network (for the edges) and a gene-level network (for the nodes). The isoforms of the same gene were collapsed into one network node. The interactions from the non-reference isoforms almost doubled the number of ASIN PPIs. Five out of seven interacting partners of the general transcription factor GTF2I were identified by screening its non-reference isoforms (inset I), whereas the majority of interacting partners of the syntaxin protein, STX1A, were identified using its reference isoform (inset II). (b) The histogram represents the number of the isoform-level PPIs (a total of 629) in ASIN coloured according to the isoform type, reference (tan) or non-reference (light blue). The Venn diagram below represents the number of the gene-level PPIs (a total of 506) in ASIN coloured according to the isoform type, reference (tan) or non-reference (light blue). Some genes have PPIs shared by the reference and the non-reference isoforms. (c) Newly identified ASIN interactions (red edges) expand known binary interactions extracted from the published literature (grey edges) by 51%. Inset I shows newly identified (red) and known (grey) interactions of the Forkhead box protein FOXP2; Inset II shows new (red) and known (grey) interactions of the T-box transcription factor TBX6 and RNA-binding protein A2BP1. (d) Alternatively spliced isoforms of A2BP1 protein and their interaction partners. Primers were designed to amplify the A2BP1 ORF that uses the downstream start site (CCDS10531) of theA2BP1gene with 15 exons that could be alternatively used. The cloned A2BP1 isoforms (two isoforms have novel exon combinations) have three alternatively spliced exons, and inclusion or exclusion of specific exons influences interaction patterns of the isoforms. Alternatively spliced exon 8 (blue, chr16:7680605-7680685); exon 10a (orange, chr16: 7714931-7714970) and exon 10b (green, chr16:7721559-7721601) mediate interactions of the isoforms with different binding partners. The genomic coordinates of exons correspond to hg19 assembly. The interactions (that is, edges) are a consensus of three independent experiments performed in triplicate. Figure 3: Splicing isoform interactions expand ASIN. ( a ) ASIN represented as two-component network consisting of reference isoforms PPIs (tan edges) and non-reference isoforms PPIs (blue edges). The network represents an isoform-level network (for the edges) and a gene-level network (for the nodes). The isoforms of the same gene were collapsed into one network node. The interactions from the non-reference isoforms almost doubled the number of ASIN PPIs. Five out of seven interacting partners of the general transcription factor GTF2I were identified by screening its non-reference isoforms (inset I), whereas the majority of interacting partners of the syntaxin protein, STX1A, were identified using its reference isoform (inset II). ( b ) The histogram represents the number of the isoform-level PPIs (a total of 629) in ASIN coloured according to the isoform type, reference (tan) or non-reference (light blue). The Venn diagram below represents the number of the gene-level PPIs (a total of 506) in ASIN coloured according to the isoform type, reference (tan) or non-reference (light blue). Some genes have PPIs shared by the reference and the non-reference isoforms. ( c ) Newly identified ASIN interactions (red edges) expand known binary interactions extracted from the published literature (grey edges) by 51%. Inset I shows newly identified (red) and known (grey) interactions of the Forkhead box protein FOXP2; Inset II shows new (red) and known (grey) interactions of the T-box transcription factor TBX6 and RNA-binding protein A2BP1. ( d ) Alternatively spliced isoforms of A2BP1 protein and their interaction partners. Primers were designed to amplify the A2BP1 ORF that uses the downstream start site (CCDS10531) of the A2BP1 gene with 15 exons that could be alternatively used. The cloned A2BP1 isoforms (two isoforms have novel exon combinations) have three alternatively spliced exons, and inclusion or exclusion of specific exons influences interaction patterns of the isoforms. Alternatively spliced exon 8 (blue, chr16:7680605-7680685); exon 10a (orange, chr16: 7714931-7714970) and exon 10b (green, chr16:7721559-7721601) mediate interactions of the isoforms with different binding partners. The genomic coordinates of exons correspond to hg19 assembly. The interactions (that is, edges) are a consensus of three independent experiments performed in triplicate. Full size image In addition to expanding the ‘reference’ network, new ASIN PPIs also expanded the LCI network of previously reported high-quality binary physical interactions from the published literature ( Supplementary Methods ). ASIN interactions increased the public network of interactions by 51% by adding 463 novel previously unreported physical associations ( Fig. 3c ). For some important ASD risk factors, such as forkhead box protein P2 (FOXP2) and A2BP1, the ASIN doubled and tripled the number of previously known interactions, respectively. In addition, 28% of the interactions we detected involve genes for which no interactions have been reported in the public databases, for example TBX6 and DGCR6 among the others. The mechanism by which splicing could influence PPIs and expand networks is directly related to the retention and loss of specific exons. For example, the A2BP1 gene coding for the ataxin-2 binding protein 1 has 16 coding exons, and at least five of them could be alternatively spliced. We cloned two new isoforms of A2BP1, A2BP1_A and A2BP1_B ( Fig. 3d ). When we tested different isoforms of A2BP1 for interactions, we observed significant variability in their interaction partners: only three interaction partners were shared among three isoforms, two partners were shared among two isoforms, and four partners were exclusively interacting with only one isoform ( Fig. 3d ). Further analysis demonstrated that inclusion or exclusion of specific exons is directly correlated with the observed PPI differences of the isoforms: differential usage of exon 8 influences interaction with CRX1; of exon 10a—with BHLHE40; of exon 10b—with four unique partners. These results suggest that differential exon usage by the splice variants could expand or even alter PPI networks, which may have important consequences for cellular function and disease, as was previously demonstrated for two splicing isoforms of the pyruvate kinase in cancer [31] . ASIN preys are enriched in genes from rare de novo CNVs Approximately half of autism risk factors (that is, ASIN baits) selected for this study are located within rare de novo or recurrent CNVs that have been identified in the patients, with many of them conferring high risk for ASD ( Supplementary Data 1 ). Thus, the ASIN network contains information on protein interactions of genes from different CNV loci . We investigated whether there was evidence of genetic association with ASD among the ‘prey’ proteins, that is, the interacting partners of the ASD candidate genes that were identified by an unbiased screen against human ORFeome (~15,000 ORFs). We assembled a dataset of 198 de novo validated autism CNVs containing 2,267 genes by combining CNV discovery results from five studies [5] , [6] , [7] , [14] , [32] . Two larger networks, Human Interactome space II 2011 (HI-II-11) and literature LCI were used as controls for this analysis (Methods). We then mapped the genes from de novo CNVs to the ASIN and HI-II-11 prey space (all ASIN baits were excluded from this analysis to eliminate the apparent CNV bias of the ASD422 list). We observed a 1.5-fold enrichment of ASIN preys in genes from de novo autism CNVs compared with the HI-II-11 preys (15.5 versus 10.6%, Fisher’s exact P =0.013; Supplementary Fig. 3a , Supplementary Table 1 ). Similar significant enrichments were observed when ASIN was compared with the LCI dataset (15.5 versus 10.1%, Fisher’s exact P =0.0047), and when only brain-expressed genes from all these datasets were analysed ( Supplementary Fig. 3b , Supplementary Table 1 ). These results suggest that proteins encoded by pathogenic autism CNVs tend to physically interact with the partners from other ASD CNVs, highlighting functional connectivity between CNV risk loci in ASD. Isoform interactions contribute to de novo CNV–prey connectivity To more deeply investigate the role of preys, we prioritized them based on the number of the CNV nodes that they connect in ASIN. Our underlying hypothesis is that network prey proteins connecting greater number of genes from the pathogenic CNVs may represent more interesting targets for future studies. Thus, we performed a subsequent analysis by merging ASIN baits from the same CNVs into the CNV nodes ( Fig. 4a ). This procedure transformed ASIN into a CNV–prey network, where ASIN risk factors (baits) are replaced with 17 CNV nodes that are connected through ASIN prey partners by the isoform interactions. We also constructed 10,000 control networks with the same characteristics as ASIN but using either HI-II-11 or LCI interactions ( Supplementary Fig. 4a ). 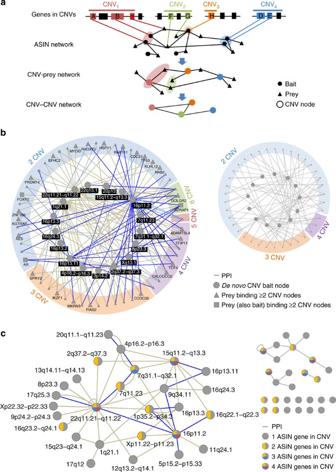Figure 4: Spliceform interactions connect genes from autism CNVs. (a) Schematic representation of the CNV–prey and CNV–CNV networks construction. The coloured horizontal bars spanning a chromosomal region represent differentde novoCNVs identified in ASD patients. Genes from the same CNVs projected (dashed coloured lines) to the ASIN network are outlined by coloured ellipses. To create a CNV–prey network, baits from the same CNVs were merged into the CNV nodes (large coloured circles) connected by the PPIs from ASIN, and baits that are not in CNVs were removed. To create a CNV–CNV network, preys were also grouped into the CNV nodes connected by the ASIN PPIs. (b) The CNV–prey network (left) identifies 26 preys (larger and darker grey triangles/squares) that bind to significantly greater number of CNV nodes than expected by chance. To identify such preys, the empiricalP-value for each prey was estimated using 10,000 degree-preserving rewired networks with exactly the same properties as ASIN. Only preys binding to ≥2 CNVs are shown. Dark blue edges are PPIs supported exclusively by the non-reference isoforms, tan edges—by the reference isoforms, light blue edges—by both isoform types. The control network (right) was selected from 10,000 control networks constructed from the randomly selected genomic regions with the same number of genes with interactions and the same number of interacting partners as in ASIN. This control network represents an example with the greatest number of preys (a total of three) that interact with four CNV nodes using HI-II-11 interactions. Among 10,000 control networks not a single network with the preys that interact with >4 CNV nodes was observed. (c) The CNV–CNV network (left) directly links 27 autism CNVs into a single connected component. Dark blue edges are PPIs supported exclusively by the non-reference isoforms, tan edges—by the reference isoforms, double edges—by both isoform types. The control network (right) represents the network that connects the largest number of CNV nodes. This network was selected from 10,000 control CNV–CNV networks constructed using randomly selected genomic regions with the same number of genes with interactions as in ASIN, connected by HI-II-11 PPIs. All networks were visualized using Cytoscape. Figure 4: Spliceform interactions connect genes from autism CNVs. ( a ) Schematic representation of the CNV–prey and CNV–CNV networks construction. The coloured horizontal bars spanning a chromosomal region represent different de novo CNVs identified in ASD patients. Genes from the same CNVs projected (dashed coloured lines) to the ASIN network are outlined by coloured ellipses. To create a CNV–prey network, baits from the same CNVs were merged into the CNV nodes (large coloured circles) connected by the PPIs from ASIN, and baits that are not in CNVs were removed. To create a CNV–CNV network, preys were also grouped into the CNV nodes connected by the ASIN PPIs. ( b ) The CNV–prey network (left) identifies 26 preys (larger and darker grey triangles/squares) that bind to significantly greater number of CNV nodes than expected by chance. To identify such preys, the empirical P -value for each prey was estimated using 10,000 degree-preserving rewired networks with exactly the same properties as ASIN. Only preys binding to ≥2 CNVs are shown. Dark blue edges are PPIs supported exclusively by the non-reference isoforms, tan edges—by the reference isoforms, light blue edges—by both isoform types. The control network (right) was selected from 10,000 control networks constructed from the randomly selected genomic regions with the same number of genes with interactions and the same number of interacting partners as in ASIN. This control network represents an example with the greatest number of preys (a total of three) that interact with four CNV nodes using HI-II-11 interactions. Among 10,000 control networks not a single network with the preys that interact with >4 CNV nodes was observed. ( c ) The CNV–CNV network (left) directly links 27 autism CNVs into a single connected component. Dark blue edges are PPIs supported exclusively by the non-reference isoforms, tan edges—by the reference isoforms, double edges—by both isoform types. The control network (right) represents the network that connects the largest number of CNV nodes. This network was selected from 10,000 control CNV–CNV networks constructed using randomly selected genomic regions with the same number of genes with interactions as in ASIN, connected by HI-II-11 PPIs. All networks were visualized using Cytoscape. Full size image We then focused our analysis on preys that link two or more CNV nodes. We observed that 26 ASIN preys interact with a significantly larger than expected number of CNV nodes and 15/26 (58%) of these preys have at least one interaction supported by a non-reference bait isoform ( Fig. 4b , Methods). For example, the majority (22/34 or 65%) of interactions that connect a high risk ASD CNV 16p11.2 in the CNV–prey network are derived exclusively from the non-reference isoforms. This suggests that isoform interactions significantly contribute to the increased CNV connectivity observed in ASIN. Two proteins, GOLGA2 and BZRAP1, linked as many as six different CNV nodes in ASIN, which is a highly unlikely event to occur by chance (empirical P <0.0001). In contrast, none of the control networks contained preys that connected more than four CNV nodes ( Supplementary Table 2 ). Two out of six PPIs of GOLGA2 and four out of six PPIs of BZRAP1 in the CNV–prey network are supported exclusively by the non-reference isoform interactions and would likely not have been detected by screening only the reference isoforms of these genes. Both genes are expressed in brain, and two recent studies have reported a de novo CNV overlapping with GOLGA2 (refs 6 , 7 ). GOLGA2 is a component of the Golgi involved in the transport of proteins and lipids, a function that is consistent with its high connectivity. BZRAP1 is a Rab3-interacting molecules (RIM)-binding protein that also binds to voltage-gated calcium channels, constituting an alternative link between RIM and calcium channels [33] . It was previously suggested as ASD risk factor in a CNV study [34] . In summary, the isoform-level PPIs support GOLGA2 and BZRAP1 as important connectors between multiple CNVs in ASIN. An isoform-resolved network directly links de novo autism CNVs We demonstrated that genes from de novo autism CNVs are connected in ASIN via prey partners. To explore whether genes from different de novo CNVs directly interact with each other at the protein level, we extended our analysis by merging both ASIN baits and preys into the CNV nodes and constructing a CNV–CNV network ( Fig. 4a ). The resulting network directly linked all 27 autism CNVs mapped to ASIN into one connected component ( Fig. 4c ). In contrast, the largest connected component of 10,000 control networks generated by permuting the locations of CNVs in the genome ranged from 1 to 12, which is significantly smaller than 27 for ASIN (empirical P <0.0001, Methods, Supplementary Fig. 4b , Supplementary Table 2 ). The CNV–CNV network directly connects proteins from several recurrent de novo CNVs (16p11.2 and 22q11.21-22; 16p11.2 and 7q31.1-q32.1; 7q31.1-q32.1 and 15q11.1-q13.3). The analysis of a more informative isoform-resolved CNV–CNV network indicates that about one third (16/47 or 34%) of the PPIs in this network are supported by the non-reference isoforms of the genes that have two or more isoforms cloned in this study ( Supplementary Fig. 5 ). More importantly, the direct CNV connections are mostly supported by novel interactions from ASIN. For example, connection between the 16p11.2 and 22q11.21-22 CNVs is supported by a novel direct interaction of Major vault protein (MVP) with RIMS-binding protein 3A (RIMBP3). Likewise, the connection between the 16p11.2 and 7q31.1-q32.1 CNVs is supported by a novel direct interaction of mitogen-activated protein kinase 3 (MAPK3) with FOXP2. A major contributor to the high connectivity of 22q11.21-q11.22 CNV, which directly links 15 other CNVs, is the DiGeorge syndrome critical region 6 protein DGCR6, for which no experimentally detected interactions have been reported before this study. ASIN provides strong support for important functional protein-level relationships between a large number of autism CNVs. The observed direct physical associations between proteins encoded by individually rare de novo CNVs points towards common molecular networks shared among different ASD patients. ASIN preys as new protein players in autism Despite a large number of preys that we have identified in ASIN (a total of 291), various types of subsequent analyses consistently highlighted a small subset of preys as being more relevant to ASD (Methods). To prioritize ASIN preys, we ranked them according to ten independent (median Pearson’s correlation coefficient (PCC)=−0.11) sources of evidence for implicating these preys in ASD ( Supplementary Fig. 6 ). A total of 31 out of 291 ASIN preys, all notably being expressed in brain, accumulated three or more sources of evidence ( Fig. 5a , Supplementary Data 6 ). Whereas 11/31 preys were previously implicated in autism, the remaining 20 are proteins that had not yet been explicitly associated with ASD at the time when this study began. Further investigation of the physical associations between highly ranked preys demonstrated that the majority of them (25/31 or 81%) interact with each other through the bait nodes that were also captured in the prey configuration in our Y2H screens ( Fig. 5b ). More importantly, 82% of the PPIs between highly ranked preys are supported exclusively by the non-reference isoforms, 12% by both, reference and non-reference isoforms and only 6% by exclusively reference isoforms. Furthermore, 58% of the PPIs are supported by the novel isoforms cloned in this study. This suggests that the majority of the interactions in this prey network would have escaped detection in the traditional reference-based PPI screens. 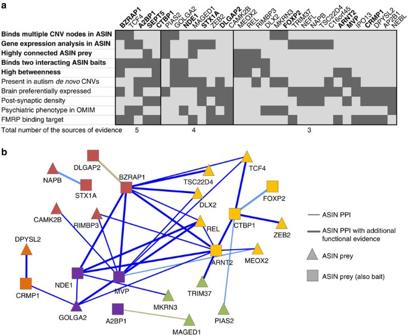Figure 5: ASIN preys as new protein players in autism. (a) Integrative analysis of ASIN implicates new players that connect autism genetic risk factors at a protein level. Ten independent sources of evidence (Methods) were used to rank ASIN preys. Thirty one preys accumulated three or more sources of independent evidence. Eleven preys (bold font) have been previously implicated in autism, whereas the remaining twenty (regular font) are newly discovered proteins with strong suggestive evidence for involvement in ASD. (b) The isoform-resolved network of binary physical interactions between highly ranked ASIN preys. Ten proteins in this network were detected in reciprocal configurations (as bait and as prey) in our Y2H screens. The majority of PPIs are supported by non-reference isoforms (dark blue lines), only two PPIs are supported by the reference isoforms (tan lines), and the remaining four by both isoform types (light blue lines). Thicker lines represent PPIs that are also supported by at least one additional functional evidence (coexpression, coregulation, co-GO annotation or complex with solved or homology-modelled structure). The network nodes are grouped according to common functional annotations of genes that were manually curated from the Genome Browser, Entrez Gene Summary and UniProt: transcription (yellow), synaptic transmission (red), cellular transport/localization (purple), SUMOylation/ubiquitination (green) and axon guidance (orange). Figure 5: ASIN preys as new protein players in autism. ( a ) Integrative analysis of ASIN implicates new players that connect autism genetic risk factors at a protein level. Ten independent sources of evidence (Methods) were used to rank ASIN preys. Thirty one preys accumulated three or more sources of independent evidence. Eleven preys (bold font) have been previously implicated in autism, whereas the remaining twenty (regular font) are newly discovered proteins with strong suggestive evidence for involvement in ASD. ( b ) The isoform-resolved network of binary physical interactions between highly ranked ASIN preys. Ten proteins in this network were detected in reciprocal configurations (as bait and as prey) in our Y2H screens. The majority of PPIs are supported by non-reference isoforms (dark blue lines), only two PPIs are supported by the reference isoforms (tan lines), and the remaining four by both isoform types (light blue lines). Thicker lines represent PPIs that are also supported by at least one additional functional evidence (coexpression, coregulation, co-GO annotation or complex with solved or homology-modelled structure). The network nodes are grouped according to common functional annotations of genes that were manually curated from the Genome Browser, Entrez Gene Summary and UniProt: transcription (yellow), synaptic transmission (red), cellular transport/localization (purple), SUMOylation/ubiquitination (green) and axon guidance (orange). Full size image While our study was in progress, some of the ASIN preys have started accumulating genetic evidence for autism relevance. For example, a highly ranked prey TCF4 was recently identified as a strong autism candidate in the whole genome sequencing of monozygotic twins [35] ; five preys ( RIMBP3, GOLGA2, MKRN3, C16orf45 and MAGED1 ) were found within newly reported de novo CNVs [6] , [7] , [14] ; and two other preys ( CASK and DISC1) were implicated in ASD based on a recent exome sequencing study [4] . Accumulating evidence suggests that many genetic risk factors are shared between different neurodevelopmental disorders [36] , [37] , [38] , [39] . We examined whether newly identified ASIN preys are involved in other neurodevelopmental syndromes characterized by psychiatric phenotypes, such as intellectual disability, mental retardation and developmental delay. We observed that ASIN is significantly enriched in preys involved in these disorders compared with HI-II-11 (5.2% versus 2.6%, Fisher’s exact P =0.02, Supplementary Table 1 , Supplementary Data 7 ), and the enrichment is maintained when analysis is restricted to only brain-expressed genes (6.1% versus 2.9%, Fisher’s exact P =0.012, Supplementary Table 1 , Supplementary Methods ). Among 31 highly ranked ASIN preys, nine are relevant to other psychiatric abnormalities (annotated as ‘psychiatric phenotype’ in Online Mendelian Inheritance in Man in Fig. 5a ). The transcription factor TCF4 is involved in Pitt-Hopkins syndrome, which is characterized by mental retardation and distinctive facial features [40] . Recently, de novo point mutations of TCF4 have been implicated in developmental delay [41] , [42] , [43] and autism [35] , and common variants of TCF4 were recurrently implicated in schizophrenia [44] , [45] . Similarly, mutations in the transcriptional inhibitor ZEB2 are the cause of Mowat–Wilson syndrome, a complex developmental disorder characterized by mental retardation, delayed motor development, epilepsy, microcephaly and a wide spectrum of clinically heterogeneous features [46] . Other psychiatric abnormalities with mutations in ASIN preys include Prader–Willi (the 15q11.2 region, which includes MKRN3 ), speech-language disorder ( FOXP2 ), and lissencephaly ( NDE1). In addition, some CNV regions harbouring highly ranked preys are associated with multiple phenotypes. For example, NDE1 is located in 16p13.11, a genomic region that is impacted by CNVs in autism [7] , [14] , schizophrenia [47] , mental retardation [48] , [49] , attention-deficit hyperactivity disorder [50] and epilepsy [51] . Considering the above observations it is tempting to speculate that the convergence of the risk factors for genetically- and phenotypically-heterogeneous neurodevelopmental disorders may occur at the level of protein interaction networks. In summary, our study emphasizes the importance of isoform-resolved PPI networks for improving understanding of autism along with other neuropsychiatric diseases. Functional relationships between genes are difficult to infer through genetic approaches alone. Our study illustrates the power of integrating genetic data with detailed isoform-resolved protein interaction network to gain better knowledge about ASD. The autism spliceform network constructed using brain-expressed gene variants is more relevant to ASD than literature-based PPI networks. ASIN has uncovered new direct physical associations between genes from pathogenic autism CNVs. It also identified new interacting partners of ASD risk factors through a large unbiased screen against thousands of other human genes. Many of the new interacting partners that we have discovered are involved in other neurodevelopmental disorders. Further functional analysis of these genes could significantly deepen our insight into pathogenesis of ASD and related disorders. ASIN is a resource with a considerable value for genetics, neurobiology and drug development. The collection of 422 cloned brain-expressed isoforms of ASD candidate genes, along with the high-quality interactome consisting of 629 isoform-based protein interactions, represents an unprecedented resource for future studies of autism. A comparison of ASIN with another recently published autism network focused on 35 syndromic autism genes [17] that does not consider interactions from the splicing isoforms, shows that these two networks are highly complementary ( Supplementary Fig. 7 ). Our study further highlights the need to include alternatively spliced isoforms of genes in future PPI screens to construct more comprehensive disease-specific and tissue-specific interactomes. It is essential to focus the disease network studies on the PPIs relevant to the tissue and pathology. Given that autism is a developmental brain disorder, the interactions identified from the brain-expressed isoforms are more appropriate for the study of ASD than PPIs from the public databases that may include interactions from the variants that are not even expressed in the human brain. Additionally, the changes in interactions of different splicing isoforms should be taken into consideration when generating and investigating disease-targeted networks. The biological relevance of a disease network is of course dependent on the disease relevance of the genes that were used to construct it. Networks built based on the findings from the genetic studies of complex diseases include a combination of true disease-associated genes and other non-relevant genes, which are expected to occur in the genetic data by chance. For example, in recent exome sequencing studies of ASD, it is estimated that only a fraction of the mutations detected in the patients (~10–20%) influence disease risk [1] , [4] . Similarly, for CNVs (even ones that have been definitively linked to ASD) only a subset of genes within the genomic region may be relevant to autism. To achieve a balance between the number of genes and the strength of evidence supporting their involvement in ASD, we decided to focus our network on the genetic variants that have strong effects, such as de novo CNVs and those implicated in the syndromic forms of ASD. In addition, we expanded the gene list with genes that have suggestive evidence, including the results of genome-wide association studies and functional studies of individual genes, to encompass a broader spectrum of the disorder. We anticipate that ASIN will be further refined as knowledge of the underlying genes contributing to ASD grows. So far, our study represents a significant step in this direction. Disease-centered networks such as ASIN could serve as valuable exploration tools for future studies. It is likely that some mutations that are currently being identified in ASD patients through exome- and whole-genome sequencing can impact or even disrupt these networks. Continued progress in genetics will rely heavily on parallel efforts to develop experimental and computational methods to distinguish between deleterious and neutral mutations. With the ASIN network constructed, we can now begin to examine how disease mutations identified in the patients impact this network, possibly through the interaction perturbation mechanisms. Furthermore, our autism spliceform network is an easily expandable resource that can keep pace with rapid advances in genetics, incorporating new findings as they emerge. Knowledge of interacting partners of ASD risk factors has direct implications for the development of therapeutics. A gene that has been firmly implicated in autism may not itself be an ideal drug target; however, an exploration of its interacting partners may identify more suitable drug targets. Selection of the autism risk factors Manually curated list of ASD risk factors was compiled in the early 2010 (before the publication of three major de novo CNV [6] , [7] , [14] and exome sequencing [1] , [2] , [3] , [4] studies) and consisted of 191 genes with suggestive evidence for involvement in ASD from earlier literature ( Supplementary Data 1 ). In assembling this list we intentionally aimed at covering as broad variety of the risk factors for non-syndromic ASD as possible, including those from different types of CNVs, which lead to the list of genes with variable degree of confidence for ASD relevance. Besides syndromic ASD risk factors (~13% of the dataset) and the genes from the de novo (~34%) and rare recurrent CNVs (~14%), the remaining candidates included genes carrying rare high penetrant mutations (~13%) and genes implicated in ASD based on other sources of evidence such as animal models, alterations in expression in the postmortem brain of ASD patients, genetic association studies and relevance to other psychiatric disorders (~26%). Brain-expressed isoform discovery pipeline The high-throughput splice isoform discovery pipeline combines high-throughput cloning and next-generation sequencing [26] . Briefly, primers corresponding to the longest-annotated ORF of each gene were designed ( Supplementary Data 8 ) and the reverse transcription was performed using the total RNA purified from the multiple pooled samples of the adult and the foetal whole normal human brains (purchased from Clontech and Stratagene). The adult brain sample contained purified whole brain RNA pooled from two healthy donors, an 18 year old male (Clontech) and a 66 year old female (Stratagene). The foetal sample contained purified whole brain RNA pooled at a 29.5:1 ratio from 59 spontaneously aborted male/female Caucasian foetuses, 20–33 w/o (Clontech), combined with two female foetuses 18 w/o (Stratagene). Reverse transcripts of brain RNAs were used as templates for the PCR amplification with KOD HotStart Polymerase (Novagen) using designed primers. Reverse transcription–PCR products were recombinationally cloned via a Gateway BP reaction (Invitrogen) with the pDONR223 vector and resulting plasmids were subsequently transformed into Escherichia coli DH5α-competent cells and grown on LB-agar plates overnight at 37 °C. A total of 32 single colonies were picked for each gene and the ORF inserts were amplified by PCR using pDONR223 universal primers (M13G forward and reverse). A total of 32 pools of PCR products were created by distributing one colony from each gene per pool and DNA products were purified using MinElute PCR Purification Kit (Qiagen). Roche 454 GS FLX sequencing was performed according to the manufacturer’s instructions. Briefly, DNA libraries were amplified from a single DNA fragment to millions of copies per bead using emulsion PCR Roche kits (GS Standard DNA Library Preparation kit; GS FLX Standard emPCR kit (Shotgun); GS FLX PicoTiterPlate Kit (70 × 75); and GS FLX Standard LR70 Sequencing Kit). Subsequent quality assessment and quantitation were performed by 96-well plate fluorometry using SpectroMax M5 (Molecular Devices) and analysed on a Bioanalyzer with Agilent RNA Pico 6000 LabChip Kit. Two 454-FLX Titanium sequencing runs (Roche) of 16 regions each were carried out at the UCSD GeneChip Microarray Core facility. Subsequently, Sanger sequencing was performed to achieve a better coverage of the 5′ and 3′ ends. Splice isoform assembly and annotation The 454 GS FLX sequencing data were assembled and analysed to identify full-length alternatively spliced ORFs using the in-house reference-based assembly pipeline ( Supplementary Fig. 1 , details in the Supplementary Methods ). In brief, raw 454 reads were processed and aligned to human genome release hg19 using GMAP [52] . Each genomic position covered by 454 reads was annotated as either exonic or intronic based on quality scores. Single-nucleotide polymorphisms and insertion/deletion (indel) variants were called using SAMtools [53] . Additional Sanger sequencing was performed to improve the assembly quality of the isoform terminal regions and was integrated using Phred [54] and CAP3 (ref. 55 ). To annotate splicing isoforms, all assembled contigs were grouped into sets of unique isoforms defined by the splicing patterns. To assess isoform novelty, unique isoform sets were compared with ORF structures of mRNAs from several major databases including CCDS, RefSeq, UCSC, Gencode (Ensembl), MGC [56] and human ORFeome [57] . Isoforms with exactly the same set of splicing sites as annotated mRNAs were considered as known, whereas isoforms with at least one novel splicing site were annotated as novel. The isoforms were translated into protein sequences using the BioPython package. All isoforms that produced short (<30 amino acid) proteins or had an out-of-frame indels within the first 20% of translated protein sequence were removed from subsequent analysis to ensure high quality of annotation. Experimental identification of PPIs The ASD422 ORFs were screened for PPIs against the human ORFeome v5.1 (~15,000 ORFs) and against themselves using a high-throughput Y2H system, retested and sequence validated ( Supplementary Fig. 2 , details in the Supplementary Methods ). First, ORFs of each isoform (Iso-ORFs) were cherry-picked from Escherichia coli glycerol stocks, cultured and cloned into pDEST-DB and pDEST-AD vectors using the Gateway recombination LR reaction (Invitrogen). Iso-ORFs in the pDEST vectors were introduced into the yeast strain Y8930 ( MATα ) to create the bait (DB-X) strains and into Y8800 ( MATa ) to create the prey (AD-Y) strains using lithium acetate transformation method. DB-X strains that autoactivated transcription of the Gal1-HIS3 reporter gene were detected and removed before the Y2H screens. The individual DB-X strains (haploid Y8930 containing Iso-ORFs in the DB vector) were screened against the pools of the AD-Y strains (haploid Y8800 containing human ORFeome v5.1 prey in the AD vector) following standard Y2H protocols [58] . Positive colonies were picked and used for making yeast lysates followed by yeast colony-PCR, stitching PCR and 454 GS FLX sequencing [59] to identify gene-level interaction pairs ( Supplementary Methods ). Isoforms of the autism risk factors were also screened against themselves (iso-ORF AD strains pooled). Four rounds of pair-wise Y2H retests among isoforms of each gene as baits and a union of all interacting partners from ORFeome 5.1/iso-ORF ADs for each gene as preys were performed in matrix format. Only the interactions that scored positive at least three times in the retests were retained. Sanger sequencing was performed to confirm ORF-level interaction pairs and to generate a high-confident isoform interactome network. Validation of Y2H interactions by MAPPIT To ensure that the interactions detected by the Y2H are of a high quality, an orthogonal assay in mammalian cells, MAPPIT [28] , [60] , was used to validate the interactions of 312 protein pairs. A random set of ASIN interactions was selected following two steps. First, 400 gene-level interacting protein pairs were randomly selected from the ASIN. Second, for those pairs where more than one isoform was interacting with the same prey, only a single isoform was randomly picked for the subsequent validation by MAPPIT. The final validation list, which consisted of 312 interaction pairs, was unique at the gene-level and comparable to the reference sets. However, interactions from the same gene were represented by different isoforms in some cases. The ASIN validation rate was compared with the validation rate of the expanded PRS consisting of ~500 positive protein pairs and the expanded RRS consisting of ~700 random protein pairs [29] , [60] using Mann–Whitney–Wilcoxon test. ASIN quality assessment using functional annotations We assessed functional similarity of interacting protein pairs using four independent measures: coexpression, coregulation, three branches of shared GO annotations and co-occurrence of interacting proteins within the same protein complex with the solved or homology-modelled protein structure. The frequencies of cofunctionally-annotated protein pairs in ASIN were compared with those from the random protein pairs set containing ~1.2 million non-redundant protein pairs generated by pairing each ASIN protein with each protein from the human ORFeome 5.1. Relative Enrichment (RE) was calculated using the given threshold (PCC ≥0.5, or 10th percentile for co-GO): where C p is the number of interacting gene pairs with coannotation above the threshold; N p is the total number of PPI pairs in a network with functional data available for both genes; C r is the number of random gene pairs with coannotation above the threshold; N r is the total number of gene pairs with functional data available for both genes. The statistical significance of the enrichment was calculated using one-tailed Fisher’s exact test. To identify coexpressed gene pairs, a publicly available human tissue expression microarray dataset was obtained from NCBI Gene Omnibus (GEO accession GSE7307) and pre-processed using robust multi-array method for background correction. Only the expression profiles from 123 healthy tissues were included; disease tissues and treated cell lines were not considered. Data filtering process was performed as follows: the probe sets with either 100% ‘absent’ calls across all tissues, or expression values <20 in all samples, or an expression range <100 across all tissues were excluded from the analysis. The expression values from replicated tissues were averaged into a single value. As a result, the expression profiles for 14,958 human genes were obtained. Gene pairs with PCC>0.5 were considered to be coexpressed. To identify coregulated gene pairs, the promoter region of each gene was defined as the region spanning 1000 base pairs upstream of the transcription start site (TSS) and 500 base pairs downstream of the TSS. RefSeq mRNA annotations were used to determine the TSS of each gene. The clustered transcriptional factor-binding sites were downloaded from the ENCODE website ( http://genome.ucsc.edu/ENCODE/ ) in BED format. Transcriptional factor-binding sites with BED scores <800 were discarded as unreliable. The gene pairs with promoter regions shared by at least one common transcription factor were considered to be coregulated. To identify co-GO-annotated gene pairs and to determine whether interacting proteins share functional similarity, we analysed annotations extracted from the GO database ( http://www.geneontology.org/GO.downloads.database.shtml ). GO annotations inferred from Electronic Annotation were excluded from the analysis as unreliable. Three GO branches (molecular function, cellular component and biological process) were used for the analyses. GO annotations were first filtered based on information content (IC). The IC of a GO term t is defined as: where p(t) is the fraction of genes annotated with the term t or its descendants. GO terms with IC< 0.95 (that is, those shared by more than 5% of all the annotated genes in one GO branch) were discarded to avoid the ‘shallow annotation problem’. After the filtering, Gene Semantic Similarity Analysis and Measurement Tools method [61] was implemented to calculate the similarity score of gene pairs in each GO branch. To identify protein pairs with solved or modelled structures, for each protein pair, the structural templates covering the interactions between domains of each protein were derived using SUPERFAMILY, DOMMINO [62] or PSI-BLAST. Once the templates were obtained, the coverage of each template was further expanded by using templates from the PDB ( http://www.pdb.org/ ). A homology model of the interaction was built using MODELLER [63] . All isoforms that participate in the interactions covered by at least one template were analysed. The same pipeline was used to assess the structural coverage of random background protein pairs. ASIN analysis using CNV data A list of 2,267 genes from the de novo validated autism CNVs was assembled by literature curation of major de novo CNV studies [5] , [6] , [7] , [14] , [32] , and a total of 69 genes from this list were successfully mapped to the ASIN. Since ASIN preys were identified using an unbiased screen against a library of ~15,000 ORFs, we used the comparable but much larger recently constructed HI-II-11 ( Supplementary Methods ) for comparison with ASIN. Both, HI-II-11 and ASIN, share the same prey search space (~15,000 ORFs), and they were both generated in the same laboratory using similar experimental conditions. Furthermore, these two networks have comparable proportions of the brain-expressed preys (85% in ASIN versus 87% in HI-II-11, Supplementary Data 9 ), making HI-II-11 the best currently available control PPI network for ASIN. The interactions from the LCI dataset were used as an additional control ( Supplementary Methods ). To construct the CNV–prey network, all baits from the same CNVs were merged into the CNV nodes. To perform statistical comparisons for Fig. 4b we generated control CNV–prey networks containing the same number of CNVs as in the ASIN CNV–prey network by randomly selecting genomic regions with the same number of genes with interactions and the same number of interacting partners as in ASIN. To ensure high quality of control networks, millions of them were generated to randomly select the sets of 10,000 networks with exactly the same parameters as ASIN CNV–preys network. Two sets of 10,000 networks each were created: one using interactions from the HI-II-11 dataset, and the other using LCI PPIs. These networks were used to estimate the statistical significance of the ASIN preys binding to multiple (≥2) unique CNVs in CNV–prey network ( Supplementary Table 2 ). The ASIN CNV–CNV network was constructed by merging both ASIN baits and preys into the CNV nodes. To perform statistical comparisons for Figure 4c we generated the sets of 10,000 control CNV–CNV networks containing the same number of CNVs as in the ASIN CNV–CNV network by randomly selecting genomic regions with the same number of genes with interactions as in ASIN. Two sets of 10,000 networks each were created: one using interactions from the HI-II-11 dataset, and the other using LCI PPIs. These networks were used to estimate the size of the largest connected component for comparison with ASIN ( Supplementary Table 2 ). ASIN prey prioritization To prioritize ASIN preys for Figure 5a , we ranked them according to ten independent sources of evidence, five from our ASIN analyses and five from the public domain. The ASIN-based sources of evidence included: (1) preys binding to a significantly greater than expected number of ASIN baits from the de novo autism CNVs identified from the CNV–prey network (a total of 26); (2) preys significantly enriched in ‘SNARE/syntaxin binding’ and ‘transcription factor binding’ from the gene coexpression and differential expression analysis (a total of 29); (3) preys binding to a greater than expected number of ASIN baits (a total of 14); (4) preys binding to two directly interacting ASIN baits and forming network triplets (a total of 25); (5) preys with high network betweenness (a total of 22). The literature-derived sources of evidence included: (1) preys from the de novo validated autism CNVs (a total of 45); (2) preys preferentially expressed in the human brain (a total of 46); (3) preys present among post-synaptic density proteins from the human neocortex (a total of 28); (4) preys annotated with psychiatric phenotype in Online Mendelian Inheritance in Man ( Supplementary Data 7 ) (a total of 15); (5) preys representing fragile X mental retardation protein (FRMP) binding targets (a total of 21). To collect the sources of evidence we have performed additional ASIN analyses as described below. To annotate preys for the Gene expression analysis in ASIN category, the unsigned coexpression network for 205 ASIN genes with available brain expression values [12] was constructed by following the standard WGCNA procedure [64] , [65] . The pair-wise correlation matrix was computed for each gene pair, and an adjacency matrix was calculated by raising the correlation matrix to a power of 10 using the scale-free topology criterion. Modules were defined as branches of the clustering tree and were characterized based on the expression of the module eigengene (ME) or the first principle component of the module. To obtain moderately large and distinct modules, the minimum module size was set to five genes and the minimum height for merging modules at 0.25. Genes were assigned to a module if they had a high module membership (kME > 0.7). Five distinct modules were detected in ASIN, and module 1 was significantly enriched in genes with ‘SNARE/syntaxin-binding’ and ‘transcription factor-binding’ functions. To identify differentially-expressed genes that interact in ASIN, brain gene expression data from autism patients and controls for 9552 genes was obtained [12] and processed using the SAM package with the significance threshold of false discovery rate (FDR) <0.05 and fold changes >1.3. Two distinct modules of interacting proteins, downregulated and upregulated in autism cases, were detected in ASIN. Functional enrichment analyses were performed for each module from WGCNA and differential expression analyses using DAVID, and statistical significance threshold was set at P <0.05 after Benjamini–Hochberg correction for multiple comparisons. To annotate preys for the Highly-connected ASIN prey category, we compared the fraction of ASIN and HI-II-11 baits interacting with each ASIN prey that is shared between ASIN and HI-II-11. We found that 14 ASIN preys interact with greater than expected number of baits (one-tailed Fisher's exact P <0.05 after false discovery rate correction). The analysis was repeated by decreasing ASIN degree or increasing HI-II-11 degree of each prey by a factor of one to ensure the robustness of the results. To annotate preys for the Binds two interacting ASIN baits category, the clustering coefficient C x of each prey x was calculated as: where N x is the number of bait neighbours of x and p x is the number of the connected pairs between all neighbours of x . To annotate preys for the High betweenness category, a modified betweenness was calculated by considering all shortest paths between ASIN baits. The betweenness of a prey (vertex) v in ASIN network graph G =( V, E ) was computed as follows: where n sd is total number of shortest paths from bait s to bait d , and n sd ( v ) is the number of the paths that traverse prey v . The betweenness of a prey v was calculated by summing B ( v ) overall pairs of vertices ( s , d ). High betweenness was defined as values in the top 25th percentile of the distribution ( B ( v )>0.027). To obtain sources of evidence from the literature, the expression profiles of 14,958 genes from 37 brain tissues and 86 other tissues (GSE7307 (ref. 66 )) were compared using a method developed by Raychaudhuri et al. [67] . A total of 2,577 genes were identified as Brain preferentially expressed with P <0.01 and 46 ASIN preys overlapped with this list. Post-synaptic density genes from the human neocortex (hPSD) (a total of 1459) were obtained from Bayés et al. [68] and 28 ASIN preys overlapped with this list. To annotate ASIN preys as FRMP-binding target, genes that are FMRP RNA targets in the mouse brain polyribosomes (a total of 839) were obtained from Darnell et al. [69] , and human orthologs of mouse genes were mapped using Mammalian Orthology from the Mouse Genome Informatics. Accession codes: Isoform nucleotide sequences have been deposited in GenBank under the accession codes KJ534756 to KJ535094 , and in the National Database for Autism Research NDAR (dataset ID: NDARCOL0001401). How to cite this article: Corominas, R. et al. Protein interaction network of alternatively spliced isoforms from brain links genetic risk factors for autism. Nat. Commun. 5:3650 doi: 10.1038/ncomms4650 (2014).